Radiation-mode optical microscopy on the growth of graphene Chemical vapour deposition (CVD) growth of graphene has attracted much attention, aiming at the mass production of large-area and high-quality specimens. To optimize the growth condition, CVD grown graphene is conventionally characterized after synthesis. Real-time observation during graphene growth enables us to understand the growth mechanism and control the growth more easily. Here we report the optical microscope observation of the CVD growth of graphene in real time by focusing the radiation emitted from the growing graphene, which we call ‘radiation-mode optical microscopy’. We observe the growth and shrinkage of graphene in response to the switching on and off of the methane supply. Analysis of the growth feature reveals that the attachment and detachment of carbon precursors are the rate-determining factor in the CVD growth of graphene. We expect radiation-mode optical microscopy to be applicable to the other crystal growth at high temperatures in various atmospheres. Chemical vapour deposition (CVD) is a film growth process in which chemical precursors decomposed from gaseous source molecules form a film on a heated substrate [1] , [2] . CVD is one of the key technologies in the semiconductor industry because of its suitability for mass production of high-quality films. In the rapidly developing field of graphene [3] , [4] and other two-dimensional (2D) materials [5] , CVD synthesis is also considered the most promising method for the scalable production of large-area and high-quality specimens [6] , [7] . In the CVD growth of graphene on Ni, for example, carbon atoms once dissolved in Ni from the source molecules segregate on the surface during the cooling process and form graphene films with a non-uniform number of layers [2] , [8] , [9] , [10] , [11] , [12] . The use of a Cu substrate with the catalytic activity and low carbon solubility, on the other hand, enables us to grow a monolayer graphene via the surface reactions of gaseous carbon source at high temperatures [1] , [2] . One of the disadvantages of the CVD process is that too many parameters to be controlled. Thus, a tremendous number of experiments are required for optimizing the growth condition and for discussing their mechanism. If the CVD process is observed in real time, it helps the optimization of parameters and the elucidation of the growth mechanism. To date, the real-time observations of the growth of graphene have been performed in ultra-high vacuum or low-pressure (<20 Pa) conditions on various metal substrates by scanning tunnelling microscopy, scanning transmission electron microscopy, low-energy electron microscopy, in situ Raman spectroscopy, environmental scanning electron microscopy (SEM) and so on [13] , [14] , [15] , [16] , [17] , [18] , [19] , [20] , [21] , [22] . From the viewpoint of scalable production of graphene, however, the combination of CH 4 gas and Cu substrate is considered the most promising, which requires the source gases with relatively high pressure from several Pa to atmospheric pressure [23] , [24] , [25] , [26] , [27] , [28] , [29] . The above-mentioned techniques could not be used for the growth of graphene on Cu under the atmosphere of source gases. Thus, the growth parameters for the Cu-CH 4 system have still been optimized generally on the basis of ‘post-synthesis’ observation with SEM, Raman spectroscopy, etc. Here we report a radiation-mode optical microscopy (Rad-OM) for in situ and real-time observation on the CVD growth of graphene on Cu from CH 4 . At the high temperatures at which graphene grows by CVD, the thermal radiation light is strong even in the visible light region [30] . Owing to the difference in the radiation intensity between Cu and graphene, the growing island of graphene is observed in real time by the instruments similar to a conventional visible–near-infrared microscope. Since the sufficient contrast can be obtained at the temperatures characteristic of the CVD growth of graphene on Cu from CH 4 , we evaluate the nucleation density, growth rate and shrinkage rate of graphene. On the basis of the temperature dependence of such growth parameters, we discuss the mechanism of the reactions that are dominated by the attachment and detachment of C precursors with graphene lattice. Rad-OM to observe graphene Optical measurements can be performed under high temperature and high pressure conditions in which graphene grows on Cu. As an example of the optical measurements on the graphene growth, in situ Raman mapping on Ni and ellipsometry on Ni and Cu were reported to observe the graphene growth in real time so far [18] , [22] . However, the microscopic optical observation has not been reported on the CVD growth on Cu. We developed the apparatus to optically observe the graphene growth in real time as shown in schematic illustration and photograph in Supplementary Figs 1 and 2 , respectively. The details of the apparatus and experiments are also described in the Methods section and in Supplementary Fig. 3 . With the present equipment, there are two ways of optical microscopic observation: reflection mode and radiation mode. When we observe the reflection from the graphene on Cu under illumination of light ( Fig. 1a ), sufficient contrast could not be obtained between graphene and Cu ( Fig. 1c ) at any temperature. At the high temperatures at which graphene grows by CVD, the material emits radiation light even in the visible light region [30] depending on its emissivity. There is a large difference in emissivity between graphite (0.8; refs 31 , 32 ) and bulk Cu (0.03; ref. 33 ) in its intrinsic state. Although it is known that the emissivity strongly depends on the flatness, chemical state of the surface and so on, the Cu substrate is flattened and reduced by the exposure to the chemically reductive molecules such as H 2 and CH 4 at high temperatures before and during the growth. Therefore, the graphene (that is, monolayer graphite) is expected to emit much radiation than the Cu substrate ( Fig. 1b ) in visible–infrared region ( Supplementary Fig. 4 ) even though the emissivity of monolayer graphene is small [34] , [35] , [36] . 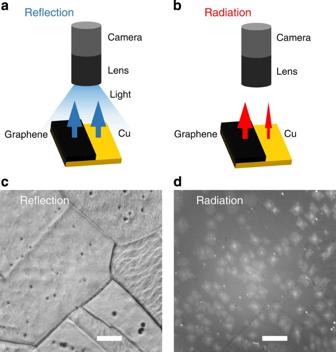Figure 1: Principle of reflection-mode and Rad-OM with apparatus. (a,b) Schematic illustrations. When the graphene on Cu is illuminated by light, the reflection intensity from the graphene on Cu is hardly different from that of a bare Cu substrate (a) due to the transparency of graphene. In contrast, the thermal radiation emitted from the graphene at high temperatures is much larger than that from Cu owing to the significant difference in their emissivities (b). (c) Reflection mode optical microscopic image obtained for graphene on Cu at 900 °C. The contrast between graphene and Cu was not observed while the surface morphology of the Cu substrate such as roughness and grain boundary can be recognized. (d) Rad-OM image obtained for graphene on Cu at 750 °C for same area as (c). The exposure time was 10 s for the image. Bright patches correspond to the graphene grains as explained inFig. 2. Scale bar, 50μm. Figure 1: Principle of reflection-mode and Rad-OM with apparatus. ( a , b ) Schematic illustrations. When the graphene on Cu is illuminated by light, the reflection intensity from the graphene on Cu is hardly different from that of a bare Cu substrate ( a ) due to the transparency of graphene. In contrast, the thermal radiation emitted from the graphene at high temperatures is much larger than that from Cu owing to the significant difference in their emissivities ( b ). ( c ) Reflection mode optical microscopic image obtained for graphene on Cu at 900 °C. The contrast between graphene and Cu was not observed while the surface morphology of the Cu substrate such as roughness and grain boundary can be recognized. ( d ) Rad-OM image obtained for graphene on Cu at 750 °C for same area as ( c ). The exposure time was 10 s for the image. Bright patches correspond to the graphene grains as explained in Fig. 2 . Scale bar, 50μm. Full size image Figure 1c,d compares the optical images of graphene on Cu between the reflection mode and radiation mode observed in real time. The spatial resolution is evaluated theoretically to be 1,800 nm, which is close to the value read in the experimentally observed height profile of the radiation intensity (see Methods section and Supplementary Fig. 5 ). In the Rad-OM image ( Fig. 1d ), there appear many bright patches that could be assigned to the graphene grains as explained below. In the reflection image, such bright grains could not be recognized, while the grain boundary of a Cu substrate is clearly observed. The contrast observed in Fig. 1d decreased with decreasing substrate temperature ( T s ), and instead the reflection of a stray light dominated the radiation ( Supplementary Fig. 6 ). Before discussing the growth mechanism of graphene, we have to confirm whether Rad-OM could practically monitor the graphene in real time or not. 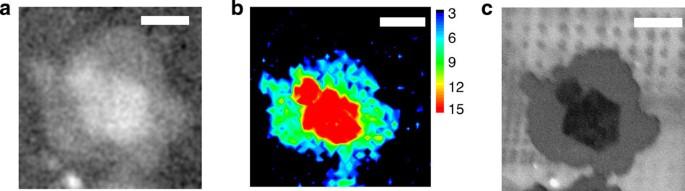Figure 2: Comparison of Rad-OM image to Raman G band intensity map and SEM image. (a) Rad-OM image of graphene on Cu substrate. The centre area (bright), periphery (grey) and surrounding area (dark) are a bilayer graphene, a monolayer graphene and the Cu substrate, respectively, (see text). (b) Raman G band intensity map indicating amount ofsp2C rings in graphene. (c) SEM image of the same grain. The centre hexagon (dark), periphery (grey) and surrounding area (white) correspond to a bilayer graphene, a monolayer graphene and the Cu substrate, respectively. Scale bar, 10μm. Figure 2a shows a typical Rad-OM image of the growing objects taken just before stopping the supply of methane. The Raman mapping of G band intensity and the SEM image of the same position are shown in Fig. 2b,c , respectively (see Methods section for post-synthesis observation). In a Raman mapping in Fig. 2b , the G band [37] intensity is large at the centre part of graphene grain as compared with the outer region. The intensity map suggested that the centre part of the graphene grain (bright region in Fig. 2a ) is a bilayer graphene and the outer part (grey region) is a monolayer graphene [38] , [39] . The fact that the outer region corresponds to a monolayer graphene was confirmed by the intensity ratio of 2D band to G band in Raman spectroscopy in Supplementary Fig. 7 . The SEM observation of many CVD graphene samples supports that the centre part (dark grey region in Fig. 2c ) was thicker than the outer region (grey) [27] . The Rad-OM image of Fig. 2a has a similar structure to those in Fig. 2b,c , while the centre part looks brighter than the outer region. It can be considered that the large amount of carbon atoms per unit area in the bilayer region emits much radiation as described in Supplementary Fig. 5 . The results in Fig. 2 proved that Rad-OM could recognize a monolayer and a bilayer graphene. The growth mechanism of graphene during the CVD process on Cu will be discussed based on the Rad-OM images in the next section. Figure 2: Comparison of Rad-OM image to Raman G band intensity map and SEM image. ( a ) Rad-OM image of graphene on Cu substrate. The centre area (bright), periphery (grey) and surrounding area (dark) are a bilayer graphene, a monolayer graphene and the Cu substrate, respectively, (see text). ( b ) Raman G band intensity map indicating amount of sp 2 C rings in graphene. ( c ) SEM image of the same grain. The centre hexagon (dark), periphery (grey) and surrounding area (white) correspond to a bilayer graphene, a monolayer graphene and the Cu substrate, respectively. Scale bar, 10μm. Full size image Real-time observation of graphene growth and shrinkage To discuss the CVD growth mechanism, we observed the growth and shrinkage processes of graphene grains on a Cu foil by Rad-OM. Growth of graphene was conducted by supplying a mixture of Ar/H 2 /CH 4 at 1,000/100/2-10 standard cubic centimetre per minutes (s.c.c.m.) under the total pressure of 2,700 Pa (see Methods section and Supplementary Fig. 3 ). 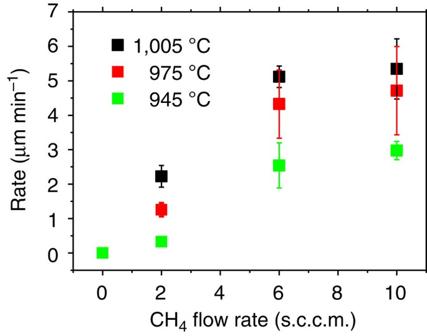Figure 3: Dependence of growth rate on CH4flow rate. The substrate temperature is 1,005, 975 and 945 °C for black, red and green squares, respectively. For each temperature, the growth rate increased with the CH4flow rate from 0 to 6 s.c.c.m. while only slightly increased from 6 to 10 s.c.c.m. Figure 3 shows the graphene growth rate with various CH 4 flow rates from 2 to 10 s.c.c.m. The way to obtain the growth rate will be shown later. The growth rate increased as the CH 4 flow rate increased from 0 to 6 s.c.c.m. at each temperature. For the CH 4 flow rate at 10 s.c.c.m., however, the growth rate increased only slightly. So we considered that 5 s.c.c.m. of CH 4 was sufficient enough to produce the precursors for the graphene growth in the present condition. The partial pressure of CH 4 under its flow rate of 5 s.c.c.m. was evaluated to be 10 Pa from the ratio of flow rates and the total pressure. 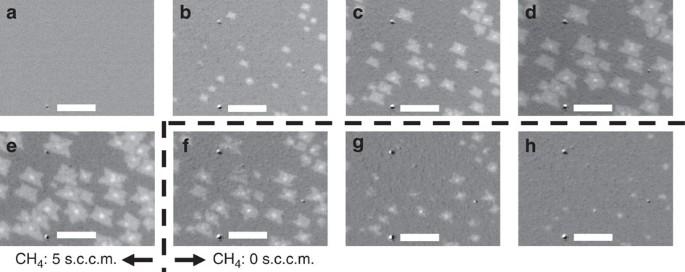Figure 4: Rad-OM images of graphene growth and shrinkage. (a–e) The growth at 0, 100, 200, 300 and 380 s with the CH4flow rate of 5 s.c.c.m. (f–h) The shrinkage at 500, 600 and 700 s with that of 0 s.c.c.m. The black dashed line is drawn to highlight the change of the CH4flow rate. All the images were picked up fromSupplementary Movie 1. Scale bar, 50μm. Figure 4 shows the images shot from the video ( Supplementary Movie 1 ) during growth with the CH 4 flow rate of 5 s.c.c.m. (0–380 s) and shrinkage without the CH 4 flow (380–700 s) at T s of 985 °C. The exposure time was 1 s, and thus the time resolution was 1 s (see Methods section). This short observation time is one of the most important characteristics of the present method. The graphene islands grew keeping their shapes as shown in Fig. 4b–e . In the following, we focus on the growth and shrinkage of a one grain of graphene to discuss the growth mechanism. If we continue the growth further beyond 380 s, graphene grains would coalesce with each other and make a continuous film covering the whole substrate, the process of which is shown in Supplementary Fig. 8 . Therefore, we stopped the growth at 380 s to assure the independent growth of each grain. The islands started to shrink after the methane supply was stopped as shown in Fig. 4f–h . It should be mentioned that the disappearance of graphene seems to occur not inside the grain but always from the periphery. In Fig. 4 , the growth of second layer graphene is also observed. The nucleation density and the growth rate seemed to be less than those of the first layer graphene. We will discuss the growth mechanism of the second layer growth later. Figure 3: Dependence of growth rate on CH 4 flow rate. The substrate temperature is 1,005, 975 and 945 °C for black, red and green squares, respectively. For each temperature, the growth rate increased with the CH 4 flow rate from 0 to 6 s.c.c.m. while only slightly increased from 6 to 10 s.c.c.m. Full size image Figure 4: Rad-OM images of graphene growth and shrinkage. ( a – e ) The growth at 0, 100, 200, 300 and 380 s with the CH 4 flow rate of 5 s.c.c.m. ( f – h ) The shrinkage at 500, 600 and 700 s with that of 0 s.c.c.m. The black dashed line is drawn to highlight the change of the CH 4 flow rate. All the images were picked up from Supplementary Movie 1 . Scale bar, 50μm. 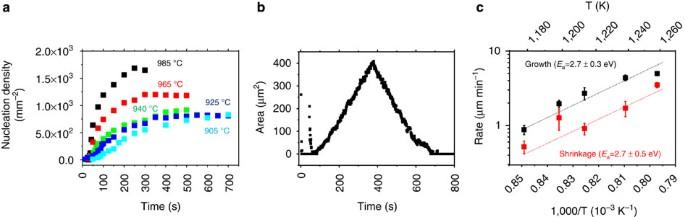Figure 5: Analysis on nucleation density and growth and shrinkage rates of graphene. (a) Time evolution of nucleation density of graphene at 985, 965, 940, 925 and 905 °C indicated as black, red, green, blue and light blue squares, respectively. (b) Time evolution of representative grain area at 985 °C. (c) Arrhenius plot of growth (black) and shrinkage (red) rates of graphene. The vertical and horizontal axis correspond to log scale of the rates and the reciprocal scale of the temperature. Activation energies (Ea) of growth and shrinkage are evaluated from the slopes to be 2.7±0.3 and 2.7±0.5 eV, respectively. Full size image Temperature dependence of graphene nucleation Figure 5a shows the evolution of the nucleation density at various T s . The saturation nucleus density ( n sat ) increases from 7.5 × 10 2 to 1.5 × 10 3 mm −2 as T s increases from 905 to 985 °C. In the previous reports, on the other hand, n sat decreased with increasing T s [26] , [27] , [28] , [29] . In physical vapour deposition, n sat usually decreases with T s because the higher T s enhances re-evaporation of source particles, leading to the decrease of surface particle density [40] . As a result, both n sat and the growth velocity tend to decrease with increasing T s . In the case of CVD growth of graphene on Cu, however, the production of precursors by dehydrogenation of methane is necessary and its activation energy is considered to be rather high [41] . The nucleation from the precursors also has a high E a of 1–4 eV (refs 26 , 27 , 28 ). Under this situation, the production of precursors and the nucleation from precursors depend strongly on T s [42] , and thus the increase in n sat with T s seems reasonable in the CVD growth of graphene [27] . The other elementary steps such as the adsorption of CH 4 to Cu surface or the surface diffusion of C precursor has lower E a [43] . Therefore, these phenomena can be excluded in the discussion about the T s dependence of growth at high temperatures. Unfortunately the present results could not be compared directly with the previous results because they were on the basis of the post-synthesis observation. We speculate about the reason of the opposite tendency as follows: (1) The growth temperature higher than 1,000 °C causes sublimation of Cu together with C precursors [28] . (2) If the growth rate increases more rapidly than the nucleation rate, the apparent nucleation density would decrease at higher temperatures. Further studies are required to reveal the temperature dependence of the nucleation density for the growth of large-area graphene. Figure 5: Analysis on nucleation density and growth and shrinkage rates of graphene. ( a ) Time evolution of nucleation density of graphene at 985, 965, 940, 925 and 905 °C indicated as black, red, green, blue and light blue squares, respectively. ( b ) Time evolution of representative grain area at 985 °C. ( c ) Arrhenius plot of growth (black) and shrinkage (red) rates of graphene. The vertical and horizontal axis correspond to log scale of the rates and the reciprocal scale of the temperature. Activation energies ( E a ) of growth and shrinkage are evaluated from the slopes to be 2.7±0.3 and 2.7±0.5 eV, respectively. Full size image Growth and shrinkage mechanism of graphene To discuss the lateral growth and shrinkage of graphene, the area of a typical graphene island at T s of 985 °C is plotted as a function of time in Fig. 5b . The ways to obtain the area of graphene grains are described in the Methods section. As shown in Supplementary Fig. 9 , the square root of the area is proportional to the elapsed time in the intermediate time period. After 250 s, the rate seems decelerated. If the growth proceeds under a constant precursor density, the square root of the area of graphene A is proportional to the elapsed time t . When the coverage of graphene on Cu substrate increases, on the other hand, the precursor production is suppressed by the decrease in the area of exposed Cu substrate and by overlap of precursor diffusion field of the adjacent graphene grains. In this case, the growth rate R g (d A 1/2 /d t ) is no longer constant. We evaluated the growth rate R g from the slope of d A 1/2 /d t for five graphene islands at various T s in the intermediate time period within which A 1/2 was proportional to the time. The R g increased from 0.9 to 5.0 μm min −1 as T s increased from 905 to 985 °C. The shrinkage rate R s was evaluated in a similar way. R s increases from 0.5 to 3.5 μm min −1 as T s increased from 905 to 985 °C. These R s values were comparable to the detachment rate of C adatoms from the graphene on Ru (0.15 μm min −1 ) at 1,070 K (ref. 44 ). The temperature dependence of R g and R s is plotted versus T −1 in Fig. 5c . Since the R g and R s increased with temperature, we consider that the chemical reactions on the substrate surface such as precursor production and incorporation of precursors at the grain periphery play an important role. Even in the case of CVD, if the precursors are formed in the gas phase such as plasma-enhanced CVD, the growth rate decreases at high temperatures [45] . From the Arrhenius plots, the activation energy E a for R g is determined to be 2.7 eV. The higher E a value than that of the precursor production [41] suggested that the incorporation process is a rate-determining factor. In the literatures by the post-synthesis observation, the activation energy of attachment of the C precursor at the periphery of the graphene grains was evaluated: 2.6 eV for Cu [26] and 2.0 eV for Ru [16] . Therefore, the incorporation of precursors to graphene is considered to be a most likely rate-determining reaction in the present growth conditions. The activation energy for R s is also evaluated to be 2.7 eV from Fig. 5c . In the shrinkage process, the C atoms were considered to detach from the graphene lattice and to desorb from the substrate, which is affected by the reaction with residual oxygen in the system [46] . (Note: it was reported that an atomic hydrogen to etch graphene is not formed on Cu [47] .) The Arrhenius plots provided almost the similar E a values for growth and shrinkage. We consider the attachment and detachment reaction of the C precursors that have different elementary reactions. For example, the precursors decomposed from CH 4 might differ from that created by the detachment. However, it seems too premature to conclude whether the attachment and detachment occurs in the same chemical reaction or not. Further investigation is necessary to explain E a of the attachment and detachment process of the precursors. Finally, we speculate about the growth mechanism of the second layer graphene. During the lateral growth of the first layer, the C precursor concentration might increase between the first layer and the Cu substrate, giving rise to the nucleation of the second layer graphene [25] . After the nucleation, however, the precursor density decreased and was kept less than that on the bare Cu substrate, resulting in the decrease in the nucleation and growth rate of second layer graphene. The currently developed Rad-OM resembles near-infrared thermography in a sense that thermal radiation emitted from the substance is spatially resolved. The resolution of near-infrared thermography was also improved by using rather short wavelength light (800–1,000 nm; ref. 48 ). While thermography acquires information on the temperature distribution of the material surface, Rad-OM distinguishes the material appearing on the topmost surface by the difference of the radiation intensity. Although the principle is very simple, it could observe the film growth under severe conditions: high temperature and atmosphere of such inflammable gases as hydrocarbon and hydrogen. We also observed the growth of graphene on the Cu substrate even under the varied O 2 partial pressure [46] . Rad-OM is applicable to the film growth at high temperatures as far as the difference in the emissivities is large enough. With respect to the Ni substrate, another popular material for the graphene growth, its emissivity ( ∼ 0.3; ref. 49 ) is less than that of graphite. Thus, the growth of graphene on Ni is expected to be observed by Rad-OM while the S/N might be less than the Cu case. We obtained the Rad-OM images of monolayer and multilayer graphenes on a Pd substrate, the contrast of which was found less owing to the smaller difference in emissivity (Pd ∼ 0.3 (ref. 50 ) and graphite 0.8) than the Cu case. In summary, we proved that Rad-OM could directly observe the growing graphene islands and shrinkage on the Cu substrate with the spatial and time resolution of 1,800 nm and 1 s, respectively. We believe that Rad-OM will open a new path to handle the growth of materials efficiently even under high temperature and atmospheric pressure conditions. Growth and shrinkage of grapheme We observed the same position of the substrate at which the graphene islands grew and shrank. A Cu foil (6 mm × 6 mm, t =50 μm, 99.99%, CU-88-83-230, Rare Metallic, Co., Ltd) welded onto a W ribbon (4 mm × 25 mm, t =35 μm, W-463242, Nilaco) was loaded in a vacuum chamber as a sample. The total pressure in the chamber was kept at 2,700 Pa by a stable gas flow of Ar (1,000 s.c.c.m.) and H 2 (100 s.c.c.m.) and evacuation with a rotary pump. The substrate was heated to the desired temperature by flowing DC current (typically 1 V and 40 A) in the W ribbon, which kept the temperature of the chamber wall almost at room temperature. This ‘cold wall’ setup suppressed the radiation from the equipment and enabled us to observe the difference in radiation from graphene and Cu. Before the growth of graphene, the Cu foil was annealed at 920 °C for 10 min in Ar/H 2 atmosphere to flatten the surface. The flow of CH 4 (5 s.c.c.m.) caused the growth of graphene, while the shutoff of the CH 4 flow did the shrinkage of graphene. After the complete disappearance of grapheme, we waited for 5 min to remove the adsorbates. Then we changed the temperature and started a new growth of graphene. To exclude the influence of an after effect, we confirmed to obtain the same result by reversing the direction of substrate temperature change. The schematic illustration of the apparatus, photograph of it and the growth sequence are shown in Supplementary Figs 1–3 , respectively. Recording facility and detection wavelength The camera (ORCA-Flash4.0 V2 C11440-22CU, Hamamatsu Photonics K. K.) recorded the whole experiments. The magnification of the zoom lens (VH-Z50L, Keyence) and the eyepiece was × 500 and × 4, respectively. The quantum efficiency of camera has a maximum 73% at 580 nm and it decreases rapidly to 5% at 1,000 nm (in the website of the company). As described in Supplementary Fig. 4a , the radiation intensity has a maximum value at the wavelength of ∼ 2,300 nm and decreases rapidly with decreasing wavelength. Taking account of the radiation intensity and quantum efficiency, the primarily detecting wavelength is considered to range from 750 to 1,000 nm ( Supplementary Fig. 4b ). The viewport is made of quartz glass. The zoom lens is made of glass and partially CaF 2 although the detailed information of the lenses is confidential in the company. These materials are transparent in the wavelengths from 750 to 1,000 nm and cut the infrared light with a wavelength longer than 2,000 nm. Thus, the detection range is mostly the same as the curve shown in Supplementary Fig. 4b . Recording videos and resolution We recorded the movie during the whole experiment. The timing of the introduction or shutoff of CH 4 can be determined independently of the recording. The elapsed time of Supplementary Movie 1 was measured after the introduction of CH 4 . The Rad-OM images are captured by ‘HCImage’, the software bundled with the camera. The typical Rad-OM image was obtained with the exposure time and colour depth of 500 ms and 16 bits, respectively. As shown in Supplementary Fig. 10 , the observed area was 324 × 324 μm 2 corresponding to 1,024 × 1,024 pixels, so that the size of pixels is 316 nm. The spatial resolution of the system was calculated by the equation d =0.61 λ/ NA (where d , λ and NA are the spatial resolution, the wavelength of observed light and the numerical aperture of the system, respectively). Although the NA value of the system is confidential in Keyence Co., we calculated NA=0.27 from the open information about the lenses. The spatial resolution d at λ =800 nm is thus calculated as 1,800 nm. The width of slope between the graphene layers in the height profile of the absolute brightness of Rad-OM image (shown in Supplementary Fig. 5 ) are 1–2 μm, which is in agreement with a value of 1,800 nm. Image processing All the processings were conducted with ‘ImageJ’, a free software for the image manipulation. To eliminate the background, we subtracted the image at 0 s from all the images and add a constant at each pixels to avoid the negative value. Then the Gauss blur ( σ =2 pixels) was applied to the whole image to enable the detection of the shape of graphene grains for ‘ImageJ’. To adjust the video size to the regulation of Nature Communications , we cropped 640 × 480 pixels images from the original one in Supplementary Fig. 10 . The area was chosen to be a good representative of the nucleation, growth and shrinkage. For the video production, we used ‘Photoshop CS6 Extended’ with H.264 codec from Adobe Systems after the subtraction of background. The video contains 800 frames corresponding to 800 s in the experiment and was compressed to 60 frames per second. In the video and images in Supplementary Movie 1 and Fig. 4 , the contrast and brightness are adjusted by ‘auto contrast’ in ‘Photoshop’. Counting the number of nuclei and area of grapheme We counted the number of nuclei by hand and eye to obtain the nucleation density because it was difficult for ‘ImageJ’ to distinguish graphene islands from the background noises in the early stage of growth. The area of graphene was estimated by ‘ImageJ’ after the ‘Threshold’ application on all of the images with auto ‘Moments’ threshold algorithm. The counting was conducted on the original images shown in Supplementary Fig. 10 , and not on the cropped images displayed in Fig. 4 and Supplementary Movie 1 . Post-synthesis observation We quenched the growth of graphene by decreasing the temperature immediately after the shutoff of CH 4 flow in the growth sequence. The ex situ measurement of Raman mapping was conducted with the laser wavelength at 532 nm and the spatial resolution of 1 μm (NRS-3000, Jasco). The G band intensity map was collected at 1,585 cm −1 . The SEM observation was carried out with the acceleration energy of 5 kV (JSM-6510, JEOL). How to cite this article: Tomo-o Terasawa and Koichiro Saiki. Radiation-mode optical microscopy on the growth of graphene. Nat. Commun . 6:6834 doi: 10.1038/ncomms7834 (2015).